Amyloid precursor protein regulates neurogenesis by antagonizing miR-574-5p in the developing cerebral cortex Amyloid precursor protein (APP) is a transmembrane glycoprotein proteolytically processed to release amyloid beta, a pathological hallmark of Alzheimer’s disease. APP is expressed throughout the developing and mature brain; however, the primary function of this protein is unknown. We previously demonstrated that APP deficiency enhances neurogenesis, but the mechanisms underlying this process are not known. Here we show that APP regulates the expression of microRNAs in the cortex and in neural progenitors, specifically repressing miR-574-5p. We also show that overexpression of miR-574-5p promotes neurogenesis, but reduces the neural progenitor pool. In contrast, the reduced expression of miR-574-5p inhibits neurogenesis and stimulates proliferation in vitro and in utero . We further demonstrate that the inhibition of miR-574-5p in APP-knockout mice rescues the phenotypes associated with APP deficiency in neurogenesis. Taken together, these results reveal a mechanism in which APP regulates the neurogenesis through miRNA-mediated post-transcriptional regulation. Amyloid precursor protein (APP) is a key molecule involved in the pathogenesis of Alzheimer’s disease [1] . Although this protein is expressed throughout the developing and adult brain, the roles of APP in neural development and neural stem cell function are not well established. We recently demonstrated that ablation of APP in mice enhances neural progenitor cells (NPCs) differentiation during embryonic development [2] . We show that NPCs from APP-knockout (KO) mice exhibit a 40–50% increase in neurogenesis compared with wild-type mice during in vitro differentiation, as shown by staining with the neuronal markers Tuj1 and MAP2 (ref. 2) [2] . However, little is known about the underlying cellular and molecular mechanisms of APP-mediated neuronal differentiation during cortical development. MicroRNAs (miRNAs) are small noncoding RNA molecules that function in the transcriptional and post-transcriptional regulation of gene expression in a variety of organisms [3] . Encoded by eukaryotic nuclear DNA, miRNAs function via base pairing with complementary sequences of mRNA molecules, typically resulting in gene silencing via translational repression or targeted degradation [4] . The role of miRNAs in neuronal development and function has been recently identified, and the specific spatiotemporal expression of these molecules is essential for brain morphogenesis and neurogenesis [5] , [6] , [7] . However, the specific miRNAs that regulate the proliferation and differentiation of neural stem cells during early cortical development are not known. Here we show that APP represses miR-574-5p in NPCs in the subventricular zone (SVZ) and cortical plate (CP) regions in the developing mouse cerebral cortex. The reduction of miR-574-5p expression enhances the proliferation of neural progenitor pool, which primarily comprises of radial glial cells (RGCs). Reduction of miR-574-5p also impedes the differentiation of RGCs into neurons and inhibits the migration of immature neurons from the SVZ to the CP in the developing neocortex. Furthermore, the inhibition of miR-574-5p in APP-KO mice rescues the phenotypes associated with APP deficiency. Taken together, our data indicates miR-574-5p as an important molecule that regulates multiple phases of neurogenesis in embryonic cortex and identifies a novel miRNA regulatory pathway underlying APP-mediated effects on neural stem cell fate. Dysregulated miRNAs in the Cortex of APP-KO mice Given the emerging regulatory role of miRNAs in stem cell proliferation and differentiation, we hypothesize that APP may control the balance between proliferation and differentiation of NPCs through the regulation of specific miRNAs. Therefore, to identify the miRNAs that are differentially regulated by APP, we performed a miRNA microarray. We compare the expression profiles of 599 mouse mmu-miRNAs obtained from the E14.5 forebrains of APP-KO mice with those obtained from wild-type (WT) control mice ( Fig. 1a ). Data are analysed by subtracting the background, and the normalization of expression was performed using a cyclic Locally Weighted Regression (LOWESS) method [8] . From this analysis, we identify a cohort of 142 differentially expressed miRNA transcripts ( P <0.01, n =3, Supplementary Data 1 ). When comparing the two groups, differentials are considered significant if the fold-change Log 2 (KO/WT)≥1.7, the t -test P -value was <0.01, n =3, the difference in fluorescence intensity between the two group means was >500 arbitrary units [9] . We applied a Log 2 (KO/WT)≥1.7 cut off to the predictions, in order to focus on the smallest number of miRNAs with the highest probability in contributing to APP-mediated neural differentiation. We observe that miR-574-5p, -574-3p, -92, -483, -1,224, -21, -9, -765 and -27b are significantly upregulated, whereas miRNAs -1265, -99a, -1275 and -15b are significantly downregulated in the APP-KO ( Fig. 1b ). We select miR-574-5p for further analysis, because this miRNA show the highest level of upregulation among identified miRNAs. 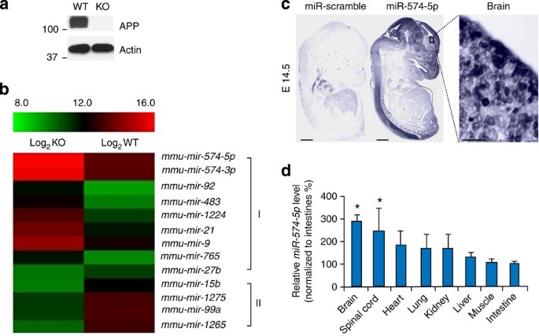Figure 1: Upregulation of miR-574-5p in the cortex of APP KO mice. (a) Western blots showing the expression of APP in WT and KO E14.5 forebrain. The full-size blot can be found inSupplementary Fig. 7. (b) A heat map of miRNAs showing the significant fold changes (log2 (KO/WT)≥1.7, thet-testP-value was <0.01,n=3) in miRNAs expression levels in the APP-KO E14.5 forebrain compared with the WT. High and low expression are denoted in red and green, respectively. The ratio values are presented in log2 format for a direct assessment of the differential direction and magnitude. Expression clusters representing different patterns of upregulation (labelled with ‘I’) to downregulation (labelled with ‘II’) are depicted with Roman numerals on the right hand side of the figure. (c) ISH was performed in an E14.5 mouse with a miR-574-5p LNA-detection probe. A sagittal section shows that miR-574-5p is expressed in the CNS. The left side section was probed with a miR-scramble control. Scale bars, 1,000 μm and 20 μm in higher magnification images. (d) Real-time PCR analyses of miR-574-5p from various tissues at E17.5, showing that miR-574-5p is highly expressed in the brain and spinal cord. The expression of miR-574-5p was measured and normalized to that of U6 and shown relative to the intestine expression level. The values represent the means±s.d. (n=3), Student’st-test, *P<0.05. Figure 1: Upregulation of miR-574-5p in the cortex of APP KO mice. ( a ) Western blots showing the expression of APP in WT and KO E14.5 forebrain. The full-size blot can be found in Supplementary Fig. 7 . ( b ) A heat map of miRNAs showing the significant fold changes (log2 (KO/WT)≥1.7, the t -test P -value was <0.01, n =3) in miRNAs expression levels in the APP-KO E14.5 forebrain compared with the WT. High and low expression are denoted in red and green, respectively. The ratio values are presented in log2 format for a direct assessment of the differential direction and magnitude. Expression clusters representing different patterns of upregulation (labelled with ‘I’) to downregulation (labelled with ‘II’) are depicted with Roman numerals on the right hand side of the figure. ( c ) ISH was performed in an E14.5 mouse with a miR-574-5p LNA-detection probe. A sagittal section shows that miR-574-5p is expressed in the CNS. The left side section was probed with a miR-scramble control. Scale bars, 1,000 μm and 20 μm in higher magnification images. ( d ) Real-time PCR analyses of miR-574-5p from various tissues at E17.5, showing that miR-574-5p is highly expressed in the brain and spinal cord. The expression of miR-574-5p was measured and normalized to that of U6 and shown relative to the intestine expression level. The values represent the means±s.d. (n=3), Student’s t -test, * P <0.05. Full size image Expression of miR-574-5p in the developing cortex We next examined the expression of miR-574-5p in the E14.5 mouse using in situ hybridization (ISH). miR-574-5p is predominately expressed in the brain and spinal cord, and no signal was detected with the scramble-miRNA probe ( Fig. 1c ). As an alternative method, we performed quantitative, real-time reserve transcription PCR (qRT–PCR) and found that miR-574-5p is expressed in a broad range of tissues; the highest expression was in the brain and spinal cord, similar to the ISH data ( Fig. 1d ). Next, we monitor the temporal expression of miR-574-5p in mouse brains during cortical development (E12.5 to postnatal day 0 (P0)). There is no detectable expression of miR-574-5p at E12.5, but we observe a gradual increase in the expression of miR-574-5p from E14.5 to P0 ( Fig. 2a ). At E14.5, miR-574-5p is highly localized in both the SVZ and the CP ( Fig. 2b ). Subsequently, we use ISH to compare miR-574-5p expression in APP-KO and WT E14.5 forebrains, which contain the SVZ and CP. We detect abundant expression of miR-574-5p in both the SVZ and CP of the WT mouse brain at E14.5 ( Fig. 2c ). In addition, we observe a more intense miR-574-5p signal in the SVZ and CP of the APP-KO brain than in the WT brain ( Fig. 2c ). We use miR-410 as a negative control as it is expressed in the mouse brain and spinal cord during CNS development [10] , and we observe that the expression of miR-410 is not differentially modulated by APP in the miRNA array analysis ( Supplementary Data 1 ). The results of the ISH study further indicate that there is no variation in the miR-410 signal intensity between the APP-KO and WT mouse brains ( Fig. 2d ). 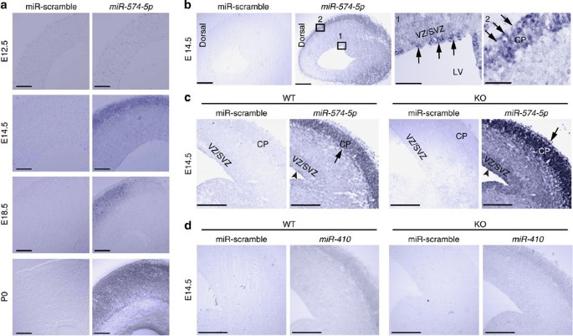Figure 2: Expression ofmiR-574-5pin the developing cortex. (a) Expression pattern ofmiR-574-5pin the developing cortex. Coronal sections of forebrain at E12.5, E14.5, E18.5 and P0 were hybridized with a miR-574-5p LNA-detection probe. The left side sections were incubated with miR-scramble control probe. Scale bars, E12.5: 100 μm; E14.5 to P0: 200 μm. (b) miR-574-5p expressed in the VZ/SVZ (1) and the CP (2) at E14.5 by ISH. Scale bars, 100 μm and 20 μm in higher magnification images (right panel). (c) ISH analysis showing the expression ofmiR-574-5pin the VZ/SVZ and the CP of E14.5 brains from WT and KO APP mice. An increased intensity signal formiR-574-5pwas observed in the APP-KO brain compared with the WT. Scale bars, 50 μm. (d) APP does not affect miR-410 expression in the VZ/SVZ and the CP area. Scale bars, 50 μm. Figure 2: Expression of miR-574-5p in the developing cortex. ( a ) Expression pattern of miR-574-5p in the developing cortex. Coronal sections of forebrain at E12.5, E14.5, E18.5 and P0 were hybridized with a miR-574-5p LNA-detection probe. The left side sections were incubated with miR-scramble control probe. Scale bars, E12.5: 100 μm; E14.5 to P0: 200 μm. ( b ) miR-574-5p expressed in the VZ/SVZ (1) and the CP (2) at E14.5 by ISH. Scale bars, 100 μm and 20 μm in higher magnification images (right panel). ( c ) ISH analysis showing the expression of miR-574-5p in the VZ/SVZ and the CP of E14.5 brains from WT and KO APP mice. An increased intensity signal for miR-574-5p was observed in the APP-KO brain compared with the WT. Scale bars, 50 μm. ( d ) APP does not affect miR-410 expression in the VZ/SVZ and the CP area. Scale bars, 50 μm. Full size image APP regulates miR-574-5p in NPCs To further determine whether APP regulates the expression of miR-574-5p , we manipulate the APP level in NPCs and measure miR-574-5p transcripts. After confirming effective knockdown of APP in vitro ( Supplementary Fig. 1 ), we use small interfering RNA (siRNA) to knockdown the expression of APP in NPCs. We then measure the level of miR-574-5p using qPCR. We find that APP knockdown upregulates miR-574-5p transcripts ( Fig. 3a ). In contrast, overexpression of APP reduces miR-574-5p transcripts ( Fig. 3b ). In addition, we overexpressed APP cDNA in NPCs from APP-KO cells and observe a similar level of miR-574-5p transcript as in WT control NPCs ( Fig. 3c ); thus, we confirm that APP-mediated miR-574-5p expression. Taken together, these data indicate that APP negatively regulates the level of miR-574-5p transcripts. To elucidate the reciprocal regulation between miR-574-5p and APP in the NPCs, we transfect NPCs with either miR-574-5p or anti-miR-574-5p and perform western blot analyses for APP. We find no change in the level of APP protein in the NPCs ( Fig. 3d ). Taken together, these data demonstrate that miR-574-5p is a downstream target of APP in NPCs. 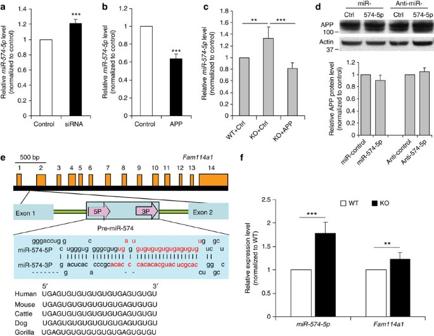Figure 3: APP regulates the expression ofmiR-574-5pin NPCs. (a) Knockdown of APP upregulatesmiR-574-5ptranscripts by qPCR assay. (b) Overexpression of APP reduced miR-574-5p transcripts. (c) Overexpression of APP in APP-KO NPCs decreases the upregulatedmiR-574-5ptranscripts. (d) Expression of miR-574-5p or anti-miR-574-5p did not affect the APP protein level by western blot. The full-size blot can be found inSupplementary Fig. 7. (e) Schematic representation of theFam114a1gene locus. miR-574-5p and -3p are generated as a stem loop encoded by the first intron ofFam114a1.Cross species conservation of miR-574-5p is shown. (f) qPCR analysis ofmiR-574-5p,Fam114a1expression in WT or APP-KO embryonic cortex. The values represent the means±s.d. (n=3). Student’st-test, ***P<0.001, **P<0.01 for all the panels in the figure. Figure 3: APP regulates the expression of miR-574-5p in NPCs. ( a ) Knockdown of APP upregulates miR-574-5p transcripts by qPCR assay. ( b ) Overexpression of APP reduced miR-574-5p transcripts. ( c ) Overexpression of APP in APP-KO NPCs decreases the upregulated miR-574-5p transcripts. ( d ) Expression of miR-574-5p or anti-miR-574-5p did not affect the APP protein level by western blot. The full-size blot can be found in Supplementary Fig. 7 . ( e ) Schematic representation of the Fam114a1 gene locus. miR-574-5p and -3p are generated as a stem loop encoded by the first intron of Fam114a1. Cross species conservation of miR-574-5p is shown. ( f ) qPCR analysis of miR-574-5p , Fam114a1 expression in WT or APP-KO embryonic cortex. The values represent the means±s.d. ( n =3). Student’s t -test, *** P <0.001, ** P <0.01 for all the panels in the figure. Full size image The gene encoding miR-574 is located in the first intron region of Fam114a1 of chromosome 5qC3.1 ( Fig. 3e ). ISH showed that Fam114a1 is highly expressed in the developing neocortex [11] . It is shown that Fam114a1 encodes Noxp20, a protein whose function may be related to early neuronal differentiation [11] . The genomic association of the two genes indicates that they may be transcriptionally co-regulated by the same set of regulatory elements and that they may be functionally correlated. Therefore, we perform qPCR of Fam114a1 from WT and APP-KO brain tissue and find that it is upregulated in the APP KO brain; Fam114a1 upregulation correlates with the expression pattern of miR-574-5p ( Fig. 3f ). This finding suggests that these two genes could be transcriptionally co-regulated by APP. miR-574-5p modulates neural differentiation To assess the potential contribution of upregulated miR-574-5p to the changes in neurogenesis, observed in the APP-KO mouse, we examine the overexpression of this miRNA in a WT animal, facilitating the separation of the contribution of miR-574-5p from other effects of APP loss in the KO. We ectopically express miR-574-5p as a short hairpin sh-miR-574-5p in NPCs isolated from the E14.5 mouse forebrain and detected a sevenfold increase in miR-574-5p expression in the transfected cells ( Supplementary Fig. 2a ). After transfection, NPCs are allowed to differentiate in vitro for 4 days by withdrawing growth factors from the culture medium. Neuronal differentiation is assayed by immunocytochemical staining with antibodies against the neuronal markers Tuj1 and MAP2. An increase in GFP and Tuj1 or MAP2 double-positive cells would indicate increased neurogenesis from NPCs, whereas a decrease in GFP and Tuj1 or MAP2 double-positive cells would indicate inhibited neurogenesis [2] . The results show that there is a 25 and 39% increase in the number of Tuj1, MAP2 and GFP double-positive cells (arrowheads), respectively, after overexpression of miR-574-5p, compared with the control vector-transfected cells ( Fig. 4a–c ). To test the loss-of-function effect of miR-574-5p in neurogenesis, we transfect NPCs with an anti-miR-574-5p-expressing vector (miR-Zip), which is designed to bind directly to miR-574-5p and inhibits its function [12] . The knockdown efficiency of miR-574-5p after transfection with miR-Zip-574-5p is confirmed by qPCR to be ~60% ( Supplementary Fig. 2b ). We observe that the number of Tuj1, MAP2 and GFP double-positive cells (arrowheads) in the miR-574-5p knockdown NPCs is 28 and 38% lower, respectively, than in the control vector-transfected cells ( Fig. 4d–f ). These data suggest that miR-574-5p positively regulates neurogenesis in vitro . 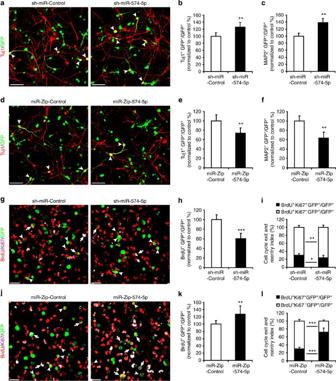Figure 4:miR-574-5p modulates the proliferation and differentiation of NPCsin vitro. (a–c) Ectopically expressed miR-574-5p (sh-miR-574-5p) in NPCs increases neurogenesis. NPCs were electroporated with plasmid expressing miR-574-5p or control vector and a neuronal differentiation assay was performed through immunostaining for Tuj1 and MAP2. The arrowheads indicate double-positive cells for Tuj1 and GFP. Scale bars, 50 μm. (d–f) NPCs transfected with miR-574-5p knockdown (miR-Zip-574-5p) show reduced neurogenesis. Scale bars, 50 μm. (g,h) Ectopically expressed miR-574-5p in NPCs reduces neural proliferation. NPCs were electroporated with plasmid expressing miR-574-5p or control vector and pulse labelled with BrdU. NPCs were immunostained with antibody against BrdU. Scale bars, 50 μm. Quantification of BrdU+GFP+cells (h). (g,i) Analysis of cell cycle exit and re-entry. NPCs were electroporated with plasmid expressing miR-574-5p or control vector and pulse labelled with BrdU. NPCs were immunostained with antibodies against BrdU and Ki67. The full arrows indicate cycling BrdU+Ki67+GFP+cells; the arrowheads indicate BrdU+Ki67−GFP+cells exiting the cell cycle. Scale bars, 50 μm. (j,k) Transfection of NPCs with anti-miR-574-5p promotes neuronal proliferation. NPCs were electroporated with miR-Zip-574-5p or control vector and pulse labelled with BrdU. NPCs were immunostained with antibody against BrdU. Scale bars, 50 μm. Quantification of BrdU+GFP+cells (k). (j,l) Analysis of cell cycle exit and re-entry. NPCs were electroporated with miR-Zip-574-5p or control vector and pulse labelled with BrdU. NPCs were immunostained with antibodies against BrdU and Ki67. The full arrows indicate cycling BrdU+Ki67+GFP+cells; the full arrows indicate BrdU+Ki67−GFP+cells exiting the cell cycle. More than 1,500 GFP-positive cells were counted for each condition. At least three sets of independent experiments were performed. The values represent the means±s.d. (n=3). Student’st-test, differences were considered significant at ***P<0.001, **P<0.01, *P<0.05. Figure 4: miR-574-5p modulates the proliferation and differentiation of NPCs in vitro . ( a – c ) Ectopically expressed miR-574-5p (sh-miR-574-5p) in NPCs increases neurogenesis. NPCs were electroporated with plasmid expressing miR-574-5p or control vector and a neuronal differentiation assay was performed through immunostaining for Tuj1 and MAP2. The arrowheads indicate double-positive cells for Tuj1 and GFP. Scale bars, 50 μm. ( d – f ) NPCs transfected with miR-574-5p knockdown (miR-Zip-574-5p) show reduced neurogenesis. Scale bars, 50 μm. ( g , h ) Ectopically expressed miR-574-5p in NPCs reduces neural proliferation. NPCs were electroporated with plasmid expressing miR-574-5p or control vector and pulse labelled with BrdU. NPCs were immunostained with antibody against BrdU. Scale bars, 50 μm. Quantification of BrdU + GFP + cells ( h ). ( g , i ) Analysis of cell cycle exit and re-entry. NPCs were electroporated with plasmid expressing miR-574-5p or control vector and pulse labelled with BrdU. NPCs were immunostained with antibodies against BrdU and Ki67. The full arrows indicate cycling BrdU + Ki67 + GFP + cells; the arrowheads indicate BrdU + Ki67 − GFP + cells exiting the cell cycle. Scale bars, 50 μm. ( j , k ) Transfection of NPCs with anti-miR-574-5p promotes neuronal proliferation. NPCs were electroporated with miR-Zip-574-5p or control vector and pulse labelled with BrdU. NPCs were immunostained with antibody against BrdU. Scale bars, 50 μm. Quantification of BrdU + GFP + cells ( k ). ( j , l ) Analysis of cell cycle exit and re-entry. NPCs were electroporated with miR-Zip-574-5p or control vector and pulse labelled with BrdU. NPCs were immunostained with antibodies against BrdU and Ki67. The full arrows indicate cycling BrdU + Ki67 + GFP + cells; the full arrows indicate BrdU + Ki67 − GFP + cells exiting the cell cycle. More than 1,500 GFP-positive cells were counted for each condition. At least three sets of independent experiments were performed. The values represent the means±s.d. ( n =3). Student’s t -test, differences were considered significant at *** P <0.001, ** P <0.01, * P <0.05. Full size image To determine whether miR-574-5p regulates the proliferation of NPCs, we examined the effect of miR-574-5p on cell proliferation using 5-bromo-2′-deoxyuridine (BrdU) pulse labelling [13] . When the cells were cultured with labelling medium containing BrdU, this pyrimidine analogue was incorporated in place of thymidine into the newly synthesized DNA of proliferating cells. We observe that the NPCs transfected with the miR-574-5p-expressing construct exhibited a 40% reduction in BrdU incorporation compared with the control vector-transfected cells, indicating that miR-574-5p inhibits NPC proliferation ( Fig. 4g,h ). In contrast, NPCs transfected with the miR-Zip-574-5p vector show a 22% increase in BrdU incorporation ( Fig. 4j,k ). To confirm the effect of miR-574-5p on neural proliferation, we performed immunostaining experiments for phosphorylated histone 3 (PH3), a mitotic marker expressed during cell cycle progression. We observe 52% fewer PH3-positive cells (arrowheads) in the miR-574-5p expression group than in the control group ( Supplementary Fig. 2c,d ) and 75% more PH3-positive cells (arrowheads) in the miR-574-5p knockdown group ( Supplementary Fig. 2e,f ). These data demonstrate that miR-574-5p inhibits the progenitor pool size. We next aim to determine the mechanism underlying the effects miR-574-5p expression on the proliferation of neural progenitors. We analyse the proliferating progenitors in more detail by performing a cell cycle exit assay [13] . We perform BrdU pulse labelling to visualize S-phase cells combined with Ki67 (ref. 14) [14] (a marker to identify all cycling cells, rather than those only in the S-phase). The percentage of BrdU and Ki67 double-positive cells is decreased in the miR-574-5p expression group ( Fig. 4g,i , arrows for BrdU + Ki67 + , and Supplementary Fig. 2g ) and elevated in the knockdown group ( Fig. 4j,l , arrows for BrdU + Ki67 + ). Conversely, the percentage of BrdU-positive and Ki67-negative cells is enhanced in the miR-574-5p expression group ( Fig. 4g,i , arrowheads for BrdU + Ki67 − ) and diminished in the miR-574-5p knockdown group ( Fig. 4j,l , arrowheads for BrdU + Ki67 − ). These data indicate that ectopic expression of miR-574-5p promotes progenitors to exit the cell cycle; in contrast, knockdown of miR-574-5p maintained cells as cycling progenitors. To determine whether cell death is affected by miR-574-5p, we knocked down or overexpressed miR-574-5p followed by TUNEL staining ( Supplementary Fig. 3a–d ) and antibody staining against active Caspase-3 ( Supplementary Fig. 3e–h ). Our results show that miR-574-5p did not affect apoptosis. miR-574-5p regulates neurogenesis in vivo To examine the effect of miR-574-5p on neural proliferation in vivo , in utero electroporation with the miR-574-5p knockdown and control vectors is performed in mice at E13.5 (ref. 13) [13] . DNA is injected into the lateral ventricular zone, and the cells lining the ventricular zone (primarily NPCs) are transfected. One day after injection, the majority of transfected cells are located at the SVZ and are immunopositive for the neural progenitor marker Sox2 ( Supplementary Fig. 4a ). In addition, there is no difference in the number of cells present in the SVZ of the control group and the miR-574-5p knockdown group ( Supplementary Fig. 4a,b ). To detect the effects of miR-574-5p on cell proliferation in vivo , coronal sections of the brain were immunostained using an antibody against the proliferation marker Ki67 at 24 h after miR-574-5p knockdown. The results of these experiments reveal a 76% increase of Ki67-positive cells (arrowheads) after miR-574-5p knockdown ( Fig. 5a,b ). Similarly, a 75% increase of PH3-positive progenitor cells (arrowheads) is detected after miR-574-5p knockdown compared with the control ( Fig. 5c,d ). Thus, the results obtained in the in vivo study are consistent with the findings from the in vitro proliferation analysis, showing that miR-574-5p inhibits NPC proliferation. 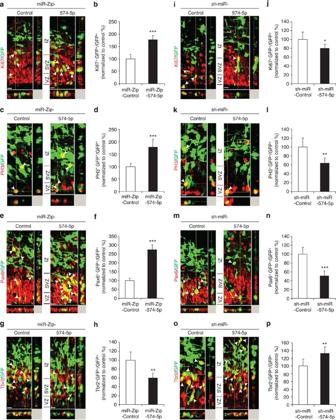Figure 5:miR-574-5p regulates RGC proliferationin vivo. Mouse embryos were electroporated at E13.5 with miR-Zip-574-5p and control vector and killed at E14.5. The brain sections were immunostained with antibodies against Ki67 (a) and PH3 (c). Scale bars, 10 μm. (b) Quantification of GFP and Ki67 double-positive cells (arrowheads) showing that miR-Zip-574-5p increases NPCs proliferation. (d) Quantification of GFP and PH3 double-positive cells (arrowheads) showing that miR-Zip-574-5p increases the number of mitotic cells. (e–h) miR-574-5p modulates the transition of RGCs to basal progenitors. Brain sections were immunostained with antibody against Pax6 (e) and Tbr2 (g). Scale bars, 10 μm. (f) Quantification of GFP and Pax6 double-positive cells (arrowheads) showing that miR-Zip-574-5p increases the RGC pool. (h) Quantification of GFP and Tbr2 double-positive cells (arrowheads) showing that miR-Zip-5745p reduces the number of basal progenitors. Overexpression of miR-574-5p followed by immunostaining with antibodies against Ki67 (i,j), PH3 (k,l), Pax6 (m,n), and Tbr2 (o,p). Scale bars, 10 μm for all panels of immunostaining. More than 1,500 GFP-positive cells were counted for each condition. At least three sets of independent experiments were performed. The values represent the means±s.d. (n=3). Student’st-test, differences were considered significant at ***P<0.001, **P<0.01, *P<0.05. Figure 5: miR-574-5p regulates RGC proliferation in vivo . Mouse embryos were electroporated at E13.5 with miR-Zip-574-5p and control vector and killed at E14.5. The brain sections were immunostained with antibodies against Ki67 ( a ) and PH3 ( c ). Scale bars, 10 μm. ( b ) Quantification of GFP and Ki67 double-positive cells (arrowheads) showing that miR-Zip-574-5p increases NPCs proliferation. ( d ) Quantification of GFP and PH3 double-positive cells (arrowheads) showing that miR-Zip-574-5p increases the number of mitotic cells. ( e – h ) miR-574-5p modulates the transition of RGCs to basal progenitors. Brain sections were immunostained with antibody against Pax6 ( e ) and Tbr2 ( g ). Scale bars, 10 μm. ( f ) Quantification of GFP and Pax6 double-positive cells (arrowheads) showing that miR-Zip-574-5p increases the RGC pool. ( h ) Quantification of GFP and Tbr2 double-positive cells (arrowheads) showing that miR-Zip-5745p reduces the number of basal progenitors. Overexpression of miR-574-5p followed by immunostaining with antibodies against Ki67 ( i , j ), PH3 ( k , l ), Pax6 ( m , n ), and Tbr2 ( o , p ). Scale bars, 10 μm for all panels of immunostaining. More than 1,500 GFP-positive cells were counted for each condition. At least three sets of independent experiments were performed. The values represent the means±s.d. ( n =3). Student’s t -test, differences were considered significant at *** P <0.001, ** P <0.01, * P <0.05. Full size image The results also demonstrate that miR-574-5p knockdown expands the VZ/SVZ progenitor pool in vivo . To gain further insight concerning how altered miR-574-5p expression affects neural cell proliferation, we electroporate E13.5 embryos with the miR-574-5p knockdown vector. One day after miRNA knockdown, we immunostain brain slices for Pax6 and Tbr2, which are markers of RGC and basal progenitor cells, respectively. We observe that the knockdown of miR-574-5p resulted in a 1.7-fold increase in Pax6-positive cells (arrowheads, Fig. 5e,f ), but 42% fewer Tbr2-positive cells (arrowheads) are observed compared with the control group ( Fig. 5g,h ). Therefore, knockdown of miR-574-5p promote neural proliferation through amplification of the RGC pool. To fully address the function of miR-574-5p in vivo , gain-of-function assays of miR-574-5p on proliferation is performed. Our results show overexpression of miR-574-5p inhibited NPC proliferation ( Fig. 5i,j for Ki67; Fig. 5k,l for PH3) and Pax6 expression ( Fig. 5m,n ) but enhanced Tbr2 ( Fig. 5o,p ). These data indicate that overexpression of miR-574-5p inhibits neural proliferation through reduction of the RGC pool. The migration of NPCs is important during the development of the embryonic nervous system and also for repair after injury in the adult brain. Tight coordination of the proliferation, migration and differentiation of NPCs is essential for the proper development of the nervous system [15] . To explore whether miR-574-5p modulates the migration of NPCs, miR-574-5p expression was knocked down in SVZ progenitor cells at E13.5 through in utero electroporation. To trace the migration process, we perform a time course measurement over the periods of 1, 2 and 4 days after electroporation. The number of transfected cells (GFP-positive) present in the VZ/SVZ, intermediate zone (IZ), and CP is quantified ( Fig. 6a–f , miR-Zip-control). At 1 day after injection (E14.5), 62% of the transfected cells are located in the VZ/SVZ ( Fig. 6a,d , miR-Zip-control). Subsequently, we observe the normal migration of electroporated cells from the ventricular zone into the IZ and CP after 2 ( Fig. 6b,e , miR-Zip-control) and 4 days ( Fig. 6c,f , miR-Zip-control). At E17.5, the cells are primarily distributed throughout the IZ and CP, with a limited number of cells remaining in the VZ/SVZ ( Fig. 6c,f , miR-Zip-control). In contrast, the miR-574-5p knockdown cells display a defect in their ability to migrate into the CP at E17.5. A majority of the miR-Zip-574-5p cells are tightly packed in the IZ and SVZ. We observed 12% of miR-574-5p knockdown cells in the CP compared with more than 25% of the control cells in the CP ( Fig. 6c,f , miR-Zip-574-5p). 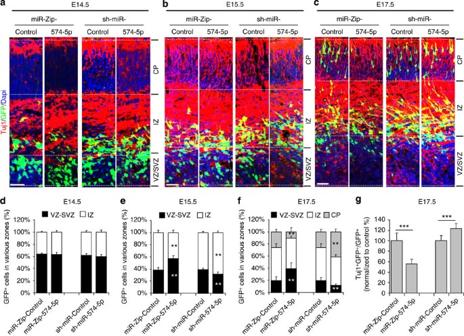Figure 6:miR-574-5p promotes the differentiation and migration of NPCsin vivo. Mouse embryos were electroporated at E13.5 to induce knockdown or overexpression of miR-574-5p or control vector and killed at E14.5 (a), E15.5 (b) and E17.5 (c). Scale bars, 20 μm. (d) Quantification of GFP-positive cells across the neocortical layers at E14.5, showing that there is no difference in the number of cells between the two groups at the VZ/SVZ and IZ. (e) Quantification of GFP-positive cells across the neocortical layers at E15.5, showing that there is an increased number of cells at the VZ/SVZ and a reduced number of cells entering the IZ in the miR-574-5p knockdown cells compared with the control group. In contrast, overexpression of miR-574-5p shows enhanced numbers of cells at the IZ. (f) Quantification of GFP-positive cells across the neocortical layers at E17.5, showing that there is a reduced number of cells entering the CP, and the majority of cells were packed at the IZ and SVZ in miR-574-5p knockdown cells. In contrast, overexpression of miR-574-5p shows increased numbers of cells entering the CP. (c,g) miR-574-5p affects neurogenesis. Brain slices were immunostained for Tuj1, and we quantified GFP and Tuj1 double-positive cells across the neocortical layers at E17.5 (c). (g) Quantification of Tuj1 and GFP-positive cells shows reduced neurogenesis in the miR-574-5p knockdown cells but enhanced neurogenesis in the miR-574-5p overexpression cells. More than 2,000 GFP-positive cells were counted for each condition. At least three sets of independent experiments were performed. The values represent the means±s.d. (n=3). Student’st-test, Differences were considered significant at ***P<0.001, **P<0.01. Figure 6: miR-574-5p promotes the differentiation and migration of NPCs in vivo . Mouse embryos were electroporated at E13.5 to induce knockdown or overexpression of miR-574-5p or control vector and killed at E14.5 ( a ), E15.5 ( b ) and E17.5 ( c ). Scale bars, 20 μm. ( d ) Quantification of GFP-positive cells across the neocortical layers at E14.5, showing that there is no difference in the number of cells between the two groups at the VZ/SVZ and IZ. ( e ) Quantification of GFP-positive cells across the neocortical layers at E15.5, showing that there is an increased number of cells at the VZ/SVZ and a reduced number of cells entering the IZ in the miR-574-5p knockdown cells compared with the control group. In contrast, overexpression of miR-574-5p shows enhanced numbers of cells at the IZ. ( f ) Quantification of GFP-positive cells across the neocortical layers at E17.5, showing that there is a reduced number of cells entering the CP, and the majority of cells were packed at the IZ and SVZ in miR-574-5p knockdown cells. In contrast, overexpression of miR-574-5p shows increased numbers of cells entering the CP. ( c , g ) miR-574-5p affects neurogenesis. Brain slices were immunostained for Tuj1, and we quantified GFP and Tuj1 double-positive cells across the neocortical layers at E17.5 ( c ). ( g ) Quantification of Tuj1 and GFP-positive cells shows reduced neurogenesis in the miR-574-5p knockdown cells but enhanced neurogenesis in the miR-574-5p overexpression cells. More than 2,000 GFP-positive cells were counted for each condition. At least three sets of independent experiments were performed. The values represent the means±s.d. ( n =3). Student’s t -test, Differences were considered significant at *** P <0.001, ** P <0.01. Full size image To assess whether miR-574-5p also regulates neurogenesis in vivo , coronal sections are immunostained using anti-Tuj1 and -GFP antibodies at E17.5. We detect a 42% reduction in the Tuj1 and GFP double-positive cells across the neocortical layers after miR-574-5p knockdown ( Fig. 6c,g , miR-Zip-574-5p). We also observe a 59% reduction in NeuN-positive cells entering the CP after transfection with the miR-Zip-574-5p compared with the control ( Supplementary Fig. 5a,b ). In contrast, overexpression of miR-574-5p promoted migration and differentiation of neurons ( Fig. 6a–f , sh-miR-574-5p for migration; Fig. 6g , sh-miR-574-5p for Tuj1). These data indicate functionally opposite effects of miR-574-5p overexpression compared with the effects of miR-574-5p knockdown. Taken together, these results suggest that miR-574-5p is important for maintaining the balance between NPCs proliferation and differentiation in vivo . In addition, miR-574-5p appears to positively regulate neuronal cell migration during cortical development. Antagonism between APP and miR-574-5p on NPCs function Our current findings and previous evidence suggest that APP and miR-574-5p might have opposite function in neural stem cells during cortical development. We next determine whether APP exerts an effect on neural differentiation through antagonism of miR-574-5p function. We transfect APP-KO NPCs with anti-miR-574-5p (miR-Zip-574-5p), as upregulation of miR-574-5p was observed in the APP-KO ( Fig. 3c ). In addition, we also express miRNA knockdown control vector in WT and APP-KO NPCs isolated from the E14.5 forebrain. We find increased neurogenesis in the APP-KO evidenced by cell staining in vitro using antibodies against Tuj1 and MAP2 (arrowheads, Fig. 7a–c , ~75 and 58% induction for Tuj1 and MAP2, respectively, compared with the control). We also notice that the knockdown of miR-574-5p in APP-KO cells reduced Tuj1- and MAP2-positive staining compared with the control vector ( Fig. 7a–c , 128 versus 175% for Tuj1; 102 versus 158% for MAP2). In addition, pulse labelling of NPCs with BrdU after miR-574-5p knockdown in APP-KO cells show enhanced proliferation of NPCs compared with APP-KO NPCs expressing the control vector ( Fig. 7d,e , 85 versus 60%). Compared with the APP WT cells, we detect a 15% increase in cell cycle exit ( Fig. 7d,f , arrowheads for BrdU + Ki67 − ) in the APP-KO NPCs combined with a decrease in cell cycle re-entry (arrows for BrdU + Ki67 + ) ( Fig. 7d,f ). Similarly, expression of miR-Zip-574-5p rescues the cell cycle deficits in APP-KO progenitor cells ( Fig. 7d,f ). 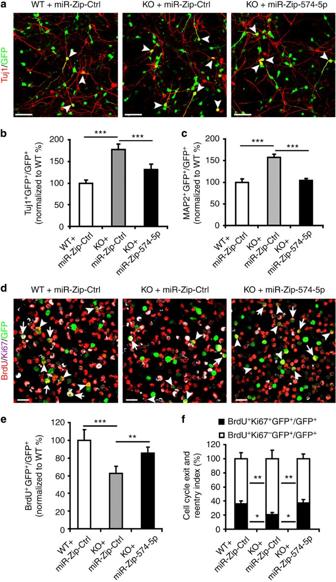Figure 7:APP antagonizes miR-574-5p-mediated NPCs functionin vitro. (a–c) APP antagonizes miR-574-5p function in neurogenesisin vitro. NPCs were isolated from E14.5 WT and KO APP embryos and electroporated with miRNA control vector. Anti-miR-574-5p (miR-Zip-574-5p) was also introduced into APP-KO NPCs to examine the rescue effect through the depletion of miR-574-5p in these cells. A neuronal differentiation assay was performed through immunostaining for Tuj1 and MAP2. Scale bars, 50 μm. The arrowheads indicate double-positive cells for Tuj1 and GFP (a). Quantification of Tuj1 (b), MAP2 (c) and GFP double-positive cells showing that knockdown of miR-5745-p in the APP-KO cells rescues enhanced neurogenesis in APP-depleted cells. (d–f) APP antagonizes miR-574-5p function in proliferationin vitro.NPCs were isolated from E14.5 WT and KO APP embryos and electroporated with miRNA control vector. Anti-miR-574-5p was also introduced into APP-KO NPCs to examine the rescue effect through the depletion of miR-574-5p in these cells. BrdU was pulse labelled, and a neural proliferation assay was performed through immunostaining for BrdU (d). Scale bars, 50 μm. (e) Quantification of BrdU and GFP double-positive cells showing that miR-574-5p knockdown in the APP-KO cells rescues the reduced proliferation in APP-depleted cells. (d,f) The knockdown of miR-574-5p rescues the cell cycle deficit in the APP-KO progenitors. Transfected NPCs were immunostained with antibodies against BrdU and Ki67. The arrows indicate cycling BrdU+Ki67+GFP+cells, and the arrowheads indicate BrdU+Ki67−GFP+cells exiting the cell cycle. Scale bars, 50 μm. More than 2,000 GFP-positive cells were counted for each condition. At least three sets of independent experiments were performed. The values represent the means±s.d. (n=3). Student’st-test, differences were considered significant at ***P<0.001, **P<0.01, *P<0.05. Figure 7: APP antagonizes miR-574-5p-mediated NPCs function in vitro . ( a – c ) APP antagonizes miR-574-5p function in neurogenesis in vitro . NPCs were isolated from E14.5 WT and KO APP embryos and electroporated with miRNA control vector. Anti-miR-574-5p (miR-Zip-574-5p) was also introduced into APP-KO NPCs to examine the rescue effect through the depletion of miR-574-5p in these cells. A neuronal differentiation assay was performed through immunostaining for Tuj1 and MAP2. Scale bars, 50 μm. The arrowheads indicate double-positive cells for Tuj1 and GFP ( a ). Quantification of Tuj1 ( b ), MAP2 ( c ) and GFP double-positive cells showing that knockdown of miR-5745-p in the APP-KO cells rescues enhanced neurogenesis in APP-depleted cells. ( d – f ) APP antagonizes miR-574-5p function in proliferation in vitro. NPCs were isolated from E14.5 WT and KO APP embryos and electroporated with miRNA control vector. Anti-miR-574-5p was also introduced into APP-KO NPCs to examine the rescue effect through the depletion of miR-574-5p in these cells. BrdU was pulse labelled, and a neural proliferation assay was performed through immunostaining for BrdU ( d ). Scale bars, 50 μm. ( e ) Quantification of BrdU and GFP double-positive cells showing that miR-574-5p knockdown in the APP-KO cells rescues the reduced proliferation in APP-depleted cells. ( d , f ) The knockdown of miR-574-5p rescues the cell cycle deficit in the APP-KO progenitors. Transfected NPCs were immunostained with antibodies against BrdU and Ki67. The arrows indicate cycling BrdU + Ki67 + GFP + cells, and the arrowheads indicate BrdU + Ki67 − GFP + cells exiting the cell cycle. Scale bars, 50 μm. More than 2,000 GFP-positive cells were counted for each condition. At least three sets of independent experiments were performed. The values represent the means±s.d. ( n =3). Student’s t -test, differences were considered significant at *** P <0.001, ** P <0.01, * P <0.05. Full size image To determine the effects of miR-574-5p on APP-mediated migration during cortical development, we electroporate E13.5 WT and KO APP cortices with the miR-574-5p knockdown or control vector. In the E17.5 APP-KO brain slice, we detect a 20% reduction of GFP-positive cells that migrated to the VZ/SVZ and IZ and an increase of GFP-positive cells in the CP compared with WT brains ( Fig. 8a,b ). The abnormal migration in the APP-KO mice is rescued by depletion of miR-574-5p ( Fig. 8a,b ). In addition, the brain slices were immunostained for Tuj1, and we count cells double-positive for Tuj1 and GFP staining across the neocortical layers. The results are consistent with the in vitro results ( Fig. 7b,c ), showing a 40% increase in neurogenesis in the APP-KO mice ( Fig. 8a,c ). Importantly, this effect is rescued by depletion of miR-574-5p in the APP-KO mice ( Fig. 8a,c ). Taken together, these results suggest that miR-574-5p serves as an important downstream effector of APP-mediated neuronal proliferation, cell cycle progression and cell migration and differentiation during cortical development. 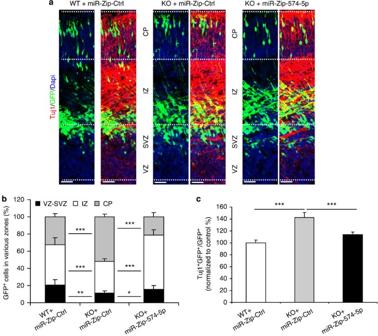Figure 8:APP antagonizes miR-574-5p-mediated migration and differentiation of NPCsin vivo. APP WT and KO mouse embryos were electroporated with miRNA control vector or anti-miR-574-5p at E13.5 and killed at E17.5. The brain sections were immunostained with antibodies against Tuj1 (a). Scale bars, 20 μm. (b) Quantification of GFP-positive cells across the neocortical layer at E17.5, showing a reduced number of cells at the IZ and an increased number of cells entering the CP in the APP-KO cells compared with WT cells. The abnormal migration defect in the APP-KO cells was further rescued through the knockdown of miR-574-5p in APP-KO mice. (c) The knockdown of miR-574-5p rescues abnormal neurogenesis in APP-depleted mice. After electroporation, the brain slices were immunostained for Tuj1, and we quantified GFP and Tuj1 double-positive cells across the neocortical layers at E17.5. More than 1,500 GFP-positive cells were counted for each condition. At least three sets of independent experiments were performed. The values represent the means±s.d. (n=3). Student’st-test, differences were considered significant at ***P<0.001, **P<0.01, *P<0.05. Figure 8: APP antagonizes miR-574-5p-mediated migration and differentiation of NPCs in vivo . APP WT and KO mouse embryos were electroporated with miRNA control vector or anti-miR-574-5p at E13.5 and killed at E17.5. The brain sections were immunostained with antibodies against Tuj1 ( a ). Scale bars, 20 μm. ( b ) Quantification of GFP-positive cells across the neocortical layer at E17.5, showing a reduced number of cells at the IZ and an increased number of cells entering the CP in the APP-KO cells compared with WT cells. The abnormal migration defect in the APP-KO cells was further rescued through the knockdown of miR-574-5p in APP-KO mice. ( c ) The knockdown of miR-574-5p rescues abnormal neurogenesis in APP-depleted mice. After electroporation, the brain slices were immunostained for Tuj1, and we quantified GFP and Tuj1 double-positive cells across the neocortical layers at E17.5. More than 1,500 GFP-positive cells were counted for each condition. At least three sets of independent experiments were performed. The values represent the means±s.d. ( n =3). Student’s t -test, differences were considered significant at *** P <0.001, ** P <0.01, * P <0.05. Full size image miR-574-5p regulates Sox12 expression in NPCs Using bioinformatics approaches [16] , [17] , we identify the top five potential miR-574-5p targets based on their functional role in neuronal development, RNA hybrid scores and the presence of synergistic binding sites [18] , [19] . These candidates are identified as Sox12, Cend1, Olig3, Dedd2 and Traf7 ( Supplementary Table 1 ). To test whether miR-574-5p targets Sox12 expression, we clone the miRNA response elements (MREs) [20] from the 3′-UTR of Sox12 into the 3′-UTR of a dual luciferase reporter construct, pmirGLO. The MREs cloned from Sox12 contained the prominent miR-574-5p seed-binding sequence ( Fig. 9a , green underlined). This allows us to assess target protein translation based on luciferase activity [20] . In this assay, SH-SY5Y cells are transfected with the plasmid constructs, and the luciferase activity was quantified after 2 days. Co-transfection of miR-574-5p with the Sox12 reporter construct suppress luciferase activity by 50% ( Fig. 9b ) compared to the control. The data indicates that the transfected miR-574-5p bound to the target MREs of Sox12 and repressed the expression of luciferase. To determine the specificity of the targeting of Sox12 by miR-574-5p, we introduce seven mismatched nucleotides in the predicted seed region of the miR-574-5p binding site ( Fig. 9a , red underline). The mismatches abolish the miR-574-5p-mediated suppression of Sox12 luciferase activity, restoring it to the control level ( Fig. 9b ). In mammals, miRNAs are shown to regulate gene expression by targeting mRNAs for degradation or by inhibiting their translation [21] . To further examine miR-574-5p-mediated repression of Sox12 at the mRNA and protein levels, we transiently over-express miR-574-5p or anti-miR-574-5p in NPCs. Indeed, we find that miR-574-5p overexpression in NPCs resulted in a reduction in both Sox12 mRNA ( Fig. 9c ) and Sox12 protein levels ( Fig. 9d ). Conversely, anti-miR-574-5p-transfected NPCs show the opposite effect on Sox12 expression ( Fig. 9c,d ). Our study suggests that miR-574-5p targets Sox12 expression in NPCs. 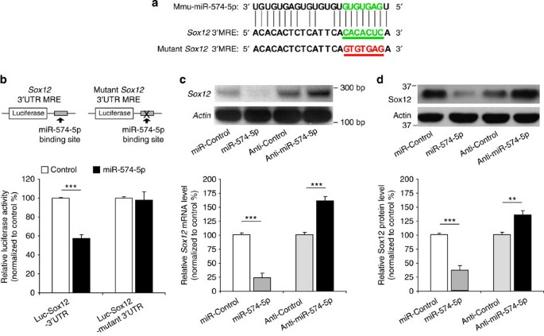Figure 9: miR-574-5p regulates Sox12 expression in NPCs. (a) TargetScan shows the miR-574-5p target site found in theSox123′-UTR region (underlined in green), and the mutantSox12(underlined in red) used in (b) is shown. (b)Sox12luciferase activity is suppressed by miR-574-5p. miR-574-5p mimic was co-transfected with the 3′-UTR ofSox12containing the miRNA-binding site in SH-SY5Y cells for 2 days. Cells were harvested and lysed, followed by a luciferase activity assay. miR-574-5p-mediated suppression ofSox12luciferase activity was released upon the mutation of the Sox12 seed-binding sites. miR-574-5p mimic was co-transfected with the mutant (MT) Sox12 binding region in SH-SY5Y cells. Cells were harvested and lysed, followed by a luciferase activity assay. (c) Overexpression of miR-574-5p in NPCs leads to reduced endogenousSox12mRNA levels by RT–PCR. Anti-miR-574-5p expression leads to increasedSox12mRNA levels. Below is the quantitative analysis. (d) miR-574-5p alters the protein expression of Sox12. Below is the quantitative analysis. Full-size blots can be found inSupplementary Fig.7. At least three sets of independent experiments were performed. Values represent the means±s.d. (n=3). Student’st-test, differences were considered significant at ***P<0.001, **P<0.01 for all panels in the figure. Figure 9: miR-574-5p regulates Sox12 expression in NPCs. ( a ) TargetScan shows the miR-574-5p target site found in the Sox12 3′-UTR region (underlined in green), and the mutant Sox12 (underlined in red) used in ( b ) is shown. ( b ) Sox12 luciferase activity is suppressed by miR-574-5p. miR-574-5p mimic was co-transfected with the 3′-UTR of Sox12 containing the miRNA-binding site in SH-SY5Y cells for 2 days. Cells were harvested and lysed, followed by a luciferase activity assay. miR-574-5p-mediated suppression of Sox12 luciferase activity was released upon the mutation of the Sox12 seed-binding sites. miR-574-5p mimic was co-transfected with the mutant (MT) Sox12 binding region in SH-SY5Y cells. Cells were harvested and lysed, followed by a luciferase activity assay. ( c ) Overexpression of miR-574-5p in NPCs leads to reduced endogenous Sox12 mRNA levels by RT–PCR. Anti-miR-574-5p expression leads to increased Sox12 mRNA levels. Below is the quantitative analysis. ( d ) miR-574-5p alters the protein expression of Sox12. Below is the quantitative analysis. Full-size blots can be found in Supplementary Fig.7 . At least three sets of independent experiments were performed. Values represent the means±s.d. ( n =3). Student’s t -test, differences were considered significant at *** P <0.001, ** P <0.01 for all panels in the figure. Full size image Next, to determine the effect of Sox12 on neurogenesis, we perform a Sox12 loss-of-function study to determine the role of Sox12 in mediating neurogenesis in NPCs. We transfected NPCs with shRNA Sox12, and differentiation is assessed by immunocytostaining with antibodies against RFP and Tuj1 ( Supplementary Fig. 6a,b ). We quantify the percentage of RFP + cells that co-expressed Tuj1 and find that neurogenesis is increased by 40% when Sox12 was knocked down ( Supplementary Fig. 6c ). The loss-of-function in Sox12 is correlated with the expression of miR-574-5p in neurogenesis, suggests that Sox12 can potentially as a downstream effector of miR-574-5p in mediating neurogenesis. APP might function as a crucial role in the regulation of neural stem cells. Here, we provide underlying mechanisms of how APP regulates the proliferation and differentiation of NPCs by controlling miR-574-5p expression. Specifically, we demonstrate that APP suppresses the expression of a brain-specific miRNA, miR-574-5p, during embryonic cortical development. High levels of miR-574-5p in NPCs promote their differentiation into neurons and inhibit the neural progenitor pool; reduced expression of miR-574-5p in NPCs has the opposite effects. Furthermore, we show that downregulation of miR-574-5p in RGCs of developing cerebral cortex promotes the amplification of the progenitor pool, which is achieved by the maintenance of cell cycle progression and inhibition of neuronal differentiation and migration. Notably, the inhibition of miR-574-5p rescues the phenotypes associated with APP deficiency ( Fig. 10 ). Our data reveal a novel mechanism in which APP controls the balance between the proliferation and differentiation of NPCs through miRNA-mediated post-transcriptional regulation. 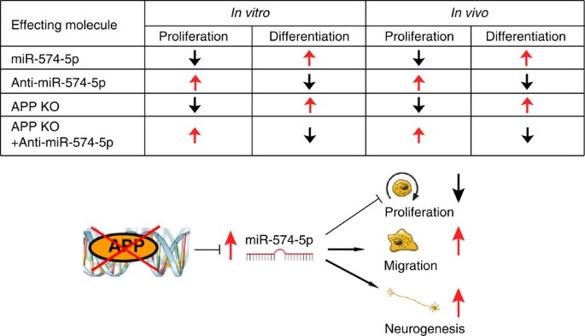Figure 10: Schematic diagram illustrating that miR-574-5p contributes to APP-mediated neural stem cell function. Our study shows that APP maintains the balance of proliferation and differentiation of NPCs; APP-KO promotes the migration and neurogenesis of NPCs but inhibits the proliferation of NPCs. Furthermore, APP suppresses the expression of miR-574-5p. Overexpression of this miRNA inhibits the proliferation of NPCs and promotes both migration and neurogenesis. Figure 10: Schematic diagram illustrating that miR-574-5p contributes to APP-mediated neural stem cell function. Our study shows that APP maintains the balance of proliferation and differentiation of NPCs; APP-KO promotes the migration and neurogenesis of NPCs but inhibits the proliferation of NPCs. Furthermore, APP suppresses the expression of miR-574-5p. Overexpression of this miRNA inhibits the proliferation of NPCs and promotes both migration and neurogenesis. Full size image Although many studies have been focused on miRNAs that regulate APP expression to Alzheimer’s disease pathogenesis [22] , [23] , [24] , we identify one of the first miRNAs (miR-574-5p) that are regulated by APP. In addition, we further suggest the mechanism of how APP regulates the transcription of miR-574-5p via regulation of transcription level of Fam114a1 , a gene which encoding miR-574-5p. Intriguingly, recent study also suggests a role of Fam114a1 in mediating early neuronal differentiation [11] . Our qPCR analysis demonstrated upregulation of Fam114a1 and miR-574-5p in the APP-KO brains ( Fig. 3 ), suggesting these two genes may be transcriptionally co-regulated by APP. We cannot exclude the relative contribution of other miRNAs that are regulated by APP, but relative abundance and spatiotemporal expression patterns of miR-574-5p suggests the importance of this miRNA during early neuronal development, when coordinated regulation of neural stem cell self-renewal and differentiation is vital for brain tissue homoeostasis [25] . Although the exact molecular mechanism of how APP-mediated regulation of miR-574-5p transcription is unclear, we speculate that APP may directly bind to the genomic regions surrounding miR-574-5p through intracellular C-terminal Domain (AICD) of APP, given that AICD can translocate to nucleus upon phosphorylation of APP and mediate some nuclear signalling events [26] , [27] , [28] . Next, what is the molecular target of miR-574-5p in regulating the proliferation and differentiation of NPCs? Our bioinformatics analysis suggests Sox12 as a potential target ( Fig. 9 , Supplementary Fig. 6 ). Sox12 is a transcription factor that shares a high degree of homology in the HMG domain and the C-terminal transactivation domain with other members like Sox4 and Sox11 in the SoxC group [29] , [30] . Sox11 has shown to be important in the transcriptional regulation of gene expression for neuronal differentiation [31] . In contrast, although Sox12 predominantly expressed in the developing human cerebral cortex and mouse neural tissue [30] , [32] , the roles of Sox12 in neural development and neural stem cell function are not clear. This could be due to the Sox12 is associated with a relatively weak transactivation efficiency in comparison with Sox11 (ref. 30) [30] . Our study may uncover the reason for the low transactivation activity observed for Sox12, which might be associated with miR-574-5p bindings. In addition, Sox12 KO mice do not show significant abnormality [29] , however, mice with double KO of Sox12 and Sox11 exhibit earlier and more widespread neurogenic defect in neural cells survival and progenitors proliferation [30] , [33] . These studies indicate that Sox12 and Sox11 may share a transcription regulatory pathway that mediates embryonic neural stem cells. Although the precise role of Sox12 in this pathway is not clear, it will be exciting to investigate whether miR-574-5p regulates embryonic neurogenesis through Sox12. Taken together, we provide experimental evidence that APP and its target miR-574-5p are important in controlling the balance between proliferation and differentiation of NPCs during vertebrate CNS development. Elucidating the mechanism by which these genes and their partners regulate cortical development will greatly enhance our understanding of APP-mediated effects on neural stem cell fate. Animals Three-month-old male and female C57BL/6 mice (National University of Singapore Comparative Medicine Centre), and 3–month-old male and female APP-KO and WT mice (Jackson Lab) were maintained in accordance with institutional guidelines, and all protocols were approved through the Institutional Animal Care and Use Committee (IACUC) of the National Neuroscience Institute, Tan Tock Seng Hospital. The mice were maintained in a pathogen-free facility and exposed to a 12-h light/dark cycle with food and water. Expression profiling of mature miRNA Approximately 10 μg of total RNA was extracted from E14.5 forebrains of WT and APP KO mice using an miRNeasy Kit (Qiagen) according to the manufacturer’s instructions. Each pair of samples was labelled with Cy3 and Cy5 fluorescent dyes and hybridized onto a single Atactic μParaFlo microfluidics chip that held 599 mature mouse mmu-miRNAs probes at the time of experiment (according to Sanger miRBase Release v.11.0 (ref. 34) [34] ). The fluorescence images were collected using a laser scanner (GenePix 4000B, CA) and digitized using Array-Pro image analysis software (Media Cybernetics, MD). Data were analysed by subtracting the background, and the normalization of expression was performed using a LOWESS method (LC Sciences). LOWESS is a pair-wise regression method that was used to normalize the samples by removing system related variations, such as sample amount variations, labelling dye differences and signal gain differences of scanners [8] . In addition, perfectly matched and mismatched probes were included on each chip for quality control of chip production, sample labelling and assay conditions. Data were analysed using analysis of variance and t -tests. When comparing the two groups, differentials were considered significant if first the fold-change Log 2 (KO/WT)≥1.7; second the t -test P -value was <0.01; and third, the difference in fluorescence intensity between the two group means was >500 arbitrary units. A heat map was generated using the log 2 -transformed values of the average signal intensities (MultiExperiment Viewer, http://www.tm4.org ). Real-time polymerase chain reaction Quantitative reverse transcription polymerase chain reaction (qRT–PCR) was performed in a quantitative manner on a Roche Light Cycler according to the manufacturer’s instructions. Total RNA, including miRNA, was isolated from tissue samples or cells using an miRNeasy kit (Qiagen). cDNA derived from 50 ng of total RNA was used directly in 20 μl real-time PCR reactions. The qRT–PCR reactions contained 1 × QuantiTect SYBR Green PCR Master mix from miScript SYBR Green PCR kit (Qiagen), 0.5 μm forward and reverse primers and nuclease-free water. U6 was used as an endogenous control for all samples. qRT–PCR was performed at 95 °C for 15 min, followed by 35 cycles at 94 °C for 15 s, 55 °C for 30 s and 70 °C for 30 s. The cycle threshold values were normalized against U6 and converted to expression abundance using the equation 2-(CTSAMPLE-CTU6). For Fam114a1 expression analysis, qRT–PCR was performed. Total RNA was isolated from tissue samples or cells using an RNeasy kit (Qiagen) followed by QuantiFast One Step qPCR. Reverse transcription was carried out at 50 °C for 10 min. PCR initial activation at 95 °C for 5 min followed by two-step cycling for 35 cycles at 95 °C for 10 s and 60 °C for 30 s. For Sox12 expression analysis, reverse transcription polymerase chain reaction (RT–PCR) was carried out. Total RNA was isolated from tissue samples or cells using an RNeasy kit (Qiagen). A total of 500 ng RNA was reverse transcribed into cDNA followed by amplification with PCR using primer pairs specific for mouse Sox12 . RT–PCR was performed at 95 °C for 1 min, 35 cycles at 95 °C for 30 s, 61 °C for 30 s, 72 °C for 40 s and a final extension step at 72 °C for 3 min. The amplified PCR products were separated on a 1.5% agarose gel, stained with ethidium bromide for visualization and photographed under ultraviolet illumination. The following primer sequences were used: mmu-miR-574-5p primer: 5′-TGAGTGTGTGTGTGTGAGTGTGT-3′. U6 forward primer: 5′-CTCGCTTCGGCAGCACA-3′, reverse primer: 5′-AACGCTTCACGAATTTGCGT-3′. Fam114a1 forward primer: 5′-CACTGTTGGGAGCAACAAGAAG-3′, reverse primer: 5′-TAGTGTCCTCAA ATGGTCTGGC-3′. Sox12 forward primer: 5′-CAGTCTGGGGACAGAGTTCC-3′, reverse primer: 5′-GACCAGTGGAGCAGACTTGG-3′. Actin forward primer: 5′-AGATGTGGATCAGCAAGCAG-3′, reverse primer: 5′-GCGCAAGTTAGGTTTTGTCA-3′. Isolation and analysis of mouse NPCs primary cultures Pregnant female animals were killed to isolate mouse embryonic E14.5 telencephalic lateral ventricle walls [2] . Tissues were digested with accutase (Innovative Cell Technologies) and cultured as neurospheres in DMEM/F12 supplemented with 10 ng ml −1 human EGF, 20 ng ml −1 human FGF2 (Invitrogen), 1% N2 supplement (GIBCO), 100 U ml −1 penicillin, 100 mg ml −1 streptomycin, and 2 mM L -glutamine in a 5% CO 2 incubator at 37 °C. The proliferation and differentiation of NPCs were performed through the early passage of the neurospheres. To study cell proliferation, we dissociated the neurospheres using accutase, followed by plating on laminin-coated glass cover-slips at a density of 20,000 cells per well. Cells were cultured in proliferation medium (see above) containing 1 μM 5-bromo-2′-deoxyuridine (BrdU, Roche). The NPCs were washed with phosphate-buffered saline and fixed with 4% paraformaldehyde for 30 min at room temperature, followed by immunocytochemical analysis. To detect BrdU incorporation, the fixed cells were pre-treated with 2 M HCl for 15 min at 37 °C, washed with borate buffer (pH 8.5) for 30 min and immunostained using a rat antibody against BrdU (#6326, Abcam). For the differentiation assay, at 24 h post-plating, the cells were changed into differentiation medium containing DMEM/F12 with 1% N2, without the growth factors FGF and EGF for 4 days. Cells were fixed with 4% paraformaldehyde for 30 min and washed with Dulbecco’s phosphate-buffered saline pH 7.4 for 30 min. The immunocytochemistry was performed after the cells were blocked using 0.1% Triton X-100 for 30 min. Cells were incubated overnight with one of the following primary antibodies (1:200): mouse anti-β III tubulin (Tuj1, #1637, Millipore), rabbit anti-Ki67 (#15580, Abcam), rabbit anti-Sox2 (#97957, Abcam), mouse anti-NueN (#MAB377, Millipore), rabbit anti-PH3 (#9701, Cell Signaling), rabbit anti-cleaved Caspase-3 (#9661, Cell Signaling), rabbit anti-Tbr2 (#23345, Abcam), rabbit anti-Pax6 (#PRB-278P, Covance). After washing with PBST, cells were incubated with secondary antibodies (1:400) that included Alexa Fluor 555 (#A31570, Invitrogen) and Alexa Fluor 488 (#A11034, Invitrogen). Cells were also counterstained with the fluorescent nuclear dye 4′,6-diamidino-2-phenylindole dihydrochloride (DAPI, Sigma-Aldrich, #B2261). For the cell apoptosis assay, TUNEL staining was performed with a kit purchased from Roche. After the cells were mounted with VECTASHIELD (VECTOR, #H-1000), the images were obtained on a confocal microscope with Olympus FV-10. Electroporation miRIDIAN miR-574-5p mimic, anti-miR-574-5p and their respective controls were obtained from Thermo Fisher Scientific. Lentiviral miR-Zip-574-5p and sh-miR-574-5p expression plasmids were obtained from System Biosciences. Human APP695 cDNA encoding sequence was first cloned from λZAP HeLa cell cDNA library and then subcloned into pcDNA3 vector (Invitrogen) at HindIII/XabI sites [35] . The FLAG sequence DYKDDDDK was inserted between APP695Ala17 and APP695Leu18 of APP695 in pcDNA3 (pAPP695NFLAG, a FLAG at the amino terminus [36] ). Four siRNAs targeting different regions of APP were purchased from GenePharma with the following sequences: 5′-GCACAUGAAUGUCCAGAAUTT-3′; 5′-CCUGCAGUAUUGCCAAGAATT-3′; 5′-CUCGUCACGUGUUCAAUAUTT-3′; 5′-GGUUCUGGGUUGACAAAUATT-3′. ShRNA Sox12: 5′-GTTCCTCCTACATACCTTA-3′ was obtained from Genecopoeia. Electroporation of these RNAs, cDNAs, shRNA and siRNAs (mix of four fragments) into NPCs was performed using a Neon electroporator (Invitrogen) according to the manufacturer’s instructions. Briefly, 1–2 × 10 6 cells were trypsinized, resuspended in Nucleofector solution, and electroporated using a preset programme for mouse NSCs. The cells were then plated onto laminin-coated 4-well plates in proliferation medium. After 24 h, the cells were changed into differentiation medium for 4 days before harvesting and fixing for the differentiation study. 3′-UTR dual luciferase assays To further study the miR-574-5p inhibition of Sox12 expression, we carried out an evaluation study on the putative miRNA recognition elements (MREs) in the 3′-UTR of Sox12 (ref. 20 ). A copy of the predicted miR-574-5p binding site was subcloned into an indicator plasmid vector pmirGLO (Promega) expressing the firefly luciferase gene. The Sox12 MRE (ACACACTCTCATTCACACACACA) was synthesized (Sense: 5′-AAACTAGCGGCCGCTAGTACACACTCTCATTCACACACACAGAGCT-3′; anti-sense: 5′-CTGTGTGTGTGAATGAGAGTGTGTACTAGCGGCCGCTAGTTT-3′), annealed and inserted into the 3′-UTR of the luc2 reporter gene at the PmeI and SacI restriction sites. Similarly, we mutated the seed region of the MRE (5′-ACACACTCTCATTGTGTGTGAGTG-3′): (Mutant MRE Sense: 5′-AAACTAGCGGCCGCTAGTACACACTCTCATTGTGTGTGAGTGAGCT-3′; anti-sense: 5′-CACTCACACACAATGAGAGTGTGTACTAGCGGCCGCTAGTTT-3′). ISH and immunohistochemistry miR-574-5p ISH detection probes was generated with a 5′-DIG-labelled locked nucleic acid detection probe (Exiqon). Embryonic brains from stages E12.5 to P0 (C57BL/6) were perfused with 4% paraformaldehyde. The brains were immersed in 30% sucrose, embedded in Tissue-Tek optimal cutting temperature compound and sectioned on the cryostat. We acetylated 12 μm coronal or 14 μm sagittal sections and treated the slices with 10 μg ml −1 Proteinase K at 37 °C for 8-15 min. After that, we pre-hybridized the slides with pre-hybridization solution for 3–4 h at 50 °C, followed by hybridization with 15 nmol locked nucleic acid digoxigenin (DIG)-labelled miRNA probes overnight at 50 °C (#K2191020, BioChain Institute, USA). The sections were then washed extensively and incubated with 1 × blocking solution for 1 h at room temperature. Subsequently, we immunostained the slides with 1:1,000 AP-conjugated anti-DIG antibody at 4 °C overnight, and washed the slides with 1 × alkaline phosphatase buffer. The signals were revealed after incubating the substrate of NBT+CIP with the slides for various times. In utero electroporation NPCs at the ventricular zone of the brain were transfected via in utero electroporation [37] . At E13.5, timed-pregnant female mice were anesthetized with ketamine/xylazine (100/10 mixture; 0.1 mg g −1 body weight, intraperitoneal injection). The uterine horns were exposed, and a lateral ventricle of each embryo was co-injected with knockdown miR-574-5p construct that was prepared by EndoFree Plasmid Maxi (3–5 μg μl −1 , Qiagen) and Fast Green (2 mg ml −1 ; Sigma-Aldrich) via a microinjector (Picospritzer III; General Valve). Approximately 1–2 μl of plasmid solution was injected into the lateral ventricle with a glass micropipette made from a microcapillary tube. Electroporation was accomplished by a BTX square wave electroporator (Harvard Apparatus) at 35 V for 50 ms on followed by 950 ms off for five pulses. The voltage was discharged across copper alloy oval plates placed on the uterine wall across the head of the embryo. Subsequently, the uterine horns were placed back into the abdominal cavity to allow the embryos to continue normal development. After electroporation, the brains were harvested at E14.5 to E17.5 and were immersed in 4% paraformaldehyde. For each plasmid injection, at least three brains were analysed. Western blotting Harvested cells were lysed in RIPA buffer containing phosphatase and protease inhibitors. Equal amounts of protein (10 μg) were separated by electrophoresis on SDS–PAGE gels and transferred onto a PVDF nitrocellulose membrane (Millipore). Membranes were probed with primary antibodies 1:1,000 (anti-Sox12, #H00006666-B01, Abnova; anti-APP, #A8717, Sigma; anti-β-actin, #SC69879, Santa Cruz) and HRP-labelled secondary antibodies 1:3,000 (#NA934V for rabbit; #NA931V for mouse, GE life Science) and visualized using an ECL kit (GE Healthcare). In vivo cell counting After in utero injection and electroporation, the mouse embryo brain was harvested and fixed with 4% paraformaldehyde and incubated in 30% sucrose overnight. A total of 15-μm coronal sections were made using a freezing microtome. For in vivo cell counting, every seven sections were collected and attached to the same glass slide, for example: No.1, 8, 15, 22. on the same glass slide. There were two advantages to use this method. First, we were able to stain the whole brain, from top to bottom, on one glass slide. Second, the interval distance between each section was at least 100 μm (15 μm × 7 sections); thus, we did not re-count the same cells in adjacent sections. After immunostaining all the sections for GFP, pictures were taken under × 20 and × 40 magnification. For the migration study, we first separated different zones by lines with DAPI staining. Subsequently, without DAPI, GFP-positive cells in different zones (lVZ-SVZ, IZ and CP) were counted and compared with total number of GFP cells on the same section. For the neurogenesis study, a Z-scan picture was taken under × 40 magnification, and the GFP and Tuj1 double-positive cells were counted and compared with the total number of GFP cells. To confirm this result, GFP and NeuN double-positive cells were also counted. Using this counting method, 1,500–2,000 GFP-positive cells were counted for each condition. At least three sets of independent experiments were performed. Statistical analysis For each experiment, at least three independent experiments were performed, and similar results were obtained. The results from one representative experiment were presented. Statistical analysis was performed using Student’s t -test. All data were presented as the mean and standard deviation of the mean (mean±s.d.). Significance was defined at *** P <0.001, ** P <0.01, * P <0.05 compared with the control. How to cite this article: Zhang, W. et al. Amyloid Precursor protein regulates neurogenesis by antagonizing miR-574-5p in the developing cerebral cortex. Nat. Commun. 5:3330 doi: 10.1038/ncomms4330 (2014).